Van der Waals negative capacitance transistors The Boltzmann distribution of electrons sets a fundamental barrier to lowering energy consumption in metal-oxide-semiconductor field-effect transistors (MOSFETs). Negative capacitance FET (NC-FET), as an emerging FET architecture, is promising to overcome this thermionic limit and build ultra-low-power consuming electronics. Here, we demonstrate steep-slope NC-FETs based on two-dimensional molybdenum disulfide and CuInP 2 S 6 (CIPS) van der Waals (vdW) heterostructure. The vdW NC-FET provides an average subthreshold swing (SS) less than the Boltzmann’s limit for over seven decades of drain current, with a minimum SS of 28 mV dec −1 . Negligible hysteresis is achieved in NC-FETs with the thickness of CIPS less than 20 nm. A voltage gain of 24 is measured for vdW NC-FET logic inverter. Flexible vdW NC-FET is further demonstrated with sub-60 mV dec −1 switching characteristics under the bending radius down to 3.8 mm. These results demonstrate the great potential of vdW NC-FET for ultra-low-power and flexible applications. Boltzmann’s limit is inevitable for traditional metal-oxide-semiconductor field-effect transistors (MOSFETs), which thermodynamically defines the lower limit of the subthreshold swing (SS) of 60 mV dec −1 at room temperature [1] , [2] , and subsequently, sets a barrier to further reduce the power consumption. Therefore, energy efficient device concepts based on scalable materials become the key to meet the great demanding in ultra-low-power applications, such as Internet-of-Things and wearable computing electronics. Negative capacitance (NC) field-effect transistor (NC-FET) has been proposed as one of the promising candidates beyond complementary metal-oxide-semiconductor (CMOS) device that may overcome the thermionic limit of 60 mV dec −1 by the internal amplification of gate voltage through ferroelectric materials [3] , [4] , [5] , [6] , [7] . Owing to their atomically thin body nature, two-dimensional (2D) transition metal dichalcogenides (TMDs) have been demonstrated to provide superior immunity to short-channel-effects [8] , [9] , [10] , [11] and suggested to achieve steep subthreshold slope over a wide voltage range for the NC-FET [12] , [13] , [14] . NC-FETs have been reported with TMDs as channel material and ferroelectric hafnium zirconium oxide (HZO) [15] , [16] , [17] or polymer [14] , [18] as ferroelectric gate. Comparing to the bulk ferroelectrics, layered ferroelectrics with atomically smooth surface may offer great performance and high reliability for NC-FETs by minimizing the dangling bonds and charged impurities induced interface traps [19] , [20] , [21] . A few 2D layered materials have been theoretically predicted or experimentally confirmed as ferroelectrics [22] , [23] , [24] , [25] . Among them, CuInP 2 S 6 (CIPS) has been shown with switchable polarization down to 4 nm at room temperature [24] . At the time of writing of this paper, Si et al. [26] reported the ferroelectric FET based on MoS 2 and CIPS heterostructure, but the sub-thermionic switching was not demonstrated due to the suspended gate structure. In this work, we demonstrate the room temperature sub-60 mV dec −1 NC-FETs using CIPS flake as the ferroelectric dielectric and atom-thin semiconductor as the channel. The average SS is less than 60 mV dec −1 for over seven decades of drain current and the minimum SS is down to 28 mV dec −1 . The hysteresis window in vdW NC-FET is suppressed by decreasing the thickness of CIPS or incorporating a thin hexagonal boron nitride (h-BN) layer into the NC gate stack. High-gain logic inverter based on vdW NC-FET is built. Bending tests show that sub-60 mV dec −1 SS can be retained and hysteresis alleviated for vdW NC-FET on polyester substrate under a bending radius down to 3.8 mm, benefiting from the intrinsic high flexibility and stretchability of 2D materials. Device design and heterostructure characterization The schematic structure of a CIPS/MoS 2 vdW NC-FET is shown in Fig. 1a , consisting of a few-layer MoS 2 as the channel material, CIPS flake and 285 nm-thick SiO 2 as the top NC and back MOS gate dielectric, respectively, heavily doped silicon substrate as the MOS gate electrode and Cr/Au as the NC gate electrode and source/drain contacts (the detailed gate-stack structure of a typical CIPS/MoS 2 vdW NC-FET is provided in Supplementary Fig. 1 ). The top-view layout of the devices is given in the false-color scanning electron microscopy (SEM) image (Fig. 1b ), where the channel length is slightly larger than the top gate length. Fig. 1 CIPS/MoS 2 vdW heterostructure and NC-FET. a , b Schematic diagram ( a ) and False-color SEM image ( b ) of a CIPS/MoS 2 vdW NC-FET. Scale bar, 2 μm. c Cross-sectional high-resolution TEM image of a vertically stacked CIPS/MoS 2 heterostructure on SiO 2 /Si substrate and corresponding EDS elemental map showing the distribution of Mo, S, Cu, In, and P. Scale bar, 5 nm. d , e PFM amplitude ( d ) and phase ( e ) of a CIPS/MoS 2 vdW heterostructure. The CIPS/MoS 2 stacked region is enclosed by dashed lines in ( d ). Scale bar, 2 μm. f The off-field PFM amplitude (top) and phase (bottom) hysteresis loops during the switching process for CIPS flake Full size image The cross-sectional transmission electron microscope (TEM) image in Fig. 1c shows the layered structure of a typical vdW ferroelectric/semiconductor heterostructure created with atomically flat CIPS and MoS 2 flakes via the dry transfer process [27] (Supplementary Note 1 and Supplementary Fig. 2 ). An atomically sharp and chemically clean interface is achieved between the vdW ferroelectric and semiconductor. The high interface quality would enable the vdW NC-FET with good performance since the NC effect is strongly correlated to interface ferroelectric domain switching. Energy-dispersive X-ray spectrometry (EDS) elemental map presented in Fig. 1c confirms the uniform distribution of Mo, S, Cu, In, and P. The ferroelectricity of CIPS was investigated using piezoresponse force microscopy (PFM) under dual AC resonance tracking (DART) mode (details about the DART mode PFM are provide in Supplementary Note 2 and Supplementary Fig. 3 and 4 ). The bright and dark regions arising from upward and downward polarizations of CIPS are clearly observed in both amplitude (Fig. 1d ) and phase (Fig. 1e ) images of local piezoresponse. The off-field PFM amplitude and phase hysteresis loops at individual point during the switching process are presented in Fig. 1f (see Supplementary Fig. 5 for the raw data). The butterfly loop in PFM amplitude and 180° phase change in the nearly square PFM phase loop confirm the good ferroelectric switching nature of CIPS. Single frequency PFM (Supplementary Fig. 6 ), polarization switching (Supplementary Fig. 7 ) and polarization versus voltage ( P - V ) hysteresis loop measurements (Supplementary Fig. 8 ) were also conducted to demonstrate the room temperature ferroelectricity in CIPS. Layer number of MoS 2 was determined by Raman spectroscopy (Supplementary Figs. 9 and 10 ). Electrical measurement of vdW NC-FETs The room temperature electrical performance of a four-layer MoS 2 device with the CIPS thickness of 51 nm, channel length of 5.7 μm and width of 5.1 μm and top gate length 3.2 μm is shown in Fig. 2a–f . Figure 2a shows the schematic of back-gate measurement configuration with 285 nm SiO 2 as the gate dielectric and top gate floating. 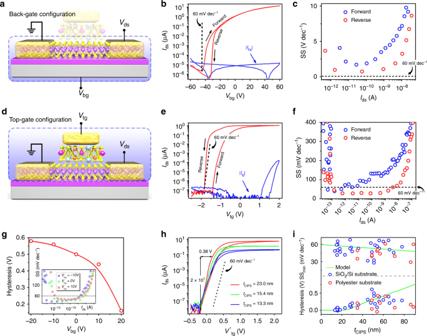Fig. 2 Room temperature electric characterization of CIPS/MoS2vdW NC-FETs.aSchematics of the characterization configuration for back-gate measurements.b,cBack-gateIds−Vbgcharacteristics (red) and leakage current (blue) (b) and SS−Idscharacteristics (c) of a CIPS/MoS2NC-FET.Vds= 0.5 V.dSchematics of the characterization configuration for top-gate measurements.e,fTop-gateIds−Vtgcharacteristics (red) and leakage current (blue) (e) and SS−Idscharacteristics (f) of the same device as in (b).gFerroelectric hysteresis dependence onVbg. Inset: SS extracted from the top-gateIds−Vtgcharacteristics at variousVbg.hTop-gate transfer characteristics of vdW NC-FETs with different thickness of CIPS.V*tg=Vtg-Vth, whereVthis the threshold voltage measured with top gate.iCIPS thickness dependence of SS (top) and hysteresis width (bottom). Symbol, experimental data; Line, simulation The I ds − V bg characteristics in Fig. 2b show a typical n-type behavior with an on/off ratio of 10 7 . The clockwise hysteresis between the forward and reverse sweeps can be attributed mainly to charge trapping at the interface of SiO 2 /MoS 2 and MOS 2 /adsorbates [28] and is suppressed to half of the original value through vacuum annealing (Supplementary Fig. 11 ). As shown in Fig. 2c , the minimum SS of MoS 2 MOSFET is derived to be 1.698 V dec −1 for forward sweep and 0.731 V dec −1 for reverse sweep according to SS = ∂ V bg /(log I ds ). Both values are far above the thermionic limit at room temperature due to the poor gate efficiency. Contrastingly, for top-gate measurement with CIPS as the ferroelectric gate insulator, so called NC-FET as illustrated in Fig. 2d , the I ds − V tg characteristics (linear scale plot of the I ds − V tg curve is provided in Supplementary Fig. 12 ) exhibit a sustained sub-60 mV dec −1 switching via the internal gate voltage amplification in NC capacitor. The conversion from clockwise hysteresis loop (Fig. 2b ) to anticlockwise one (Fig. 2e ) by top gating is a result of ferroelectric nature of CIPS and the hysteresis is found to be suppressed by reducing the V tg sweep speed (Supplementary Fig. 13 ). Compared with SiO 2 gating, the off-state current is significantly reduced in NC-FET due to the trap-free vdW interface between MoS 2 and CIPS, and the same on/off ratio is achieved despite the limited on-state current by ungated channel segments. SS extracted from the transfer characteristics of NC-FET falls below the thermionic limit for both forward and reverse sweeps, with a minimum of 39 and 28 mV dec −1 , respectively. Incompletely compensated upward polarization in CIPS due to the low hole concentration in MoS 2 leads to a larger SS for forward sweep [18] . The average SS for reverse sweep is <60 mV dec −1 for over five decades of drain current. The effectiveness of NC effect in vdW NC-FETs is also supported by the observed drain-induced-barrier-rising effect and negative-differential-resistance characteristics (Supplementary Note 3 and Supplementary Fig. 14 ), which are distinctive features not seen in the conventional MOSFETs. P-type vdW NC-FETs with sub-60 mV dec −1 SS were also demonstrated with electrically doped WSe 2 as the channel material (Supplementary Fig. 15 ). Fig. 2 Room temperature electric characterization of CIPS/MoS 2 vdW NC-FETs. a Schematics of the characterization configuration for back-gate measurements. b , c Back-gate I ds − V bg characteristics (red) and leakage current (blue) ( b ) and SS− I ds characteristics ( c ) of a CIPS/MoS 2 NC-FET. V ds = 0.5 V. d Schematics of the characterization configuration for top-gate measurements. e , f Top-gate I ds − V tg characteristics (red) and leakage current (blue) ( e ) and SS− I ds characteristics ( f ) of the same device as in ( b ). g Ferroelectric hysteresis dependence on V bg . Inset: SS extracted from the top-gate I ds − V tg characteristics at various V bg . h Top-gate transfer characteristics of vdW NC-FETs with different thickness of CIPS. V * tg = V tg - V th , where V th is the threshold voltage measured with top gate. i CIPS thickness dependence of SS (top) and hysteresis width (bottom). Symbol, experimental data; Line, simulation Full size image We then examine the impact of back-gate biasing on the top-gate transfer characteristics of NC-FET. We found that the ferroelectric hysteresis can be suppressed by positive V bg (Fig. 2g ) while the SS is slightly improved by negative V bg (inset in Fig. 2g ). We ascribe these effects to the back-gate modulation of CIPS capacitance ( C CIPS ). A vdW NC-FET can be represented as an underlying 2D FET in series with a ferroelectric CIPS capacitor. Therefore, the internal gate voltage amplification gain is derived as A V = | C CIPS |/( C CIPS | − C int ), where C int is the top-gate capacitance of underlying 2D FET. Then the SS of the vdW NCFET can be expressed as SS NCFET = SS 2DFET / A V . To obtain a large A V and small SS, C int should be very close to | C CIPS |. However, in order to avoid hysteresis, C int must be smaller than | C CIPS | [29] . The increase of underlying MoS 2 FET channel charge by applying a positive V bg leads to an increase in | C CIPS |, resulting in a reduced hysteresis and increased SS for NC-FET. Device architecture optimization Optimized vdW NC-FETs were fabricated to achieve steep switching and reduce the hysteresis by controlling the thickness of ferroelectric CIPS layer. Figure 2h shows the transfer characteristics of vdW NC-FETs with 23.0, 15.4, and 13.3 nm CIPS ( I ds – V tg characteristics of NC-FETs with 29.0 and 20.0 nm CIPS are provided in Supplementary Fig. 16 ). A minimum SS of 41.8 mV dec −1 for reverse sweep with a hysteresis of 70 mV at I ds = 10 pA is achieved for 23.0 nm CIPS, less than the one of 453 mV for 51.0 nm CIPS shown in Fig. 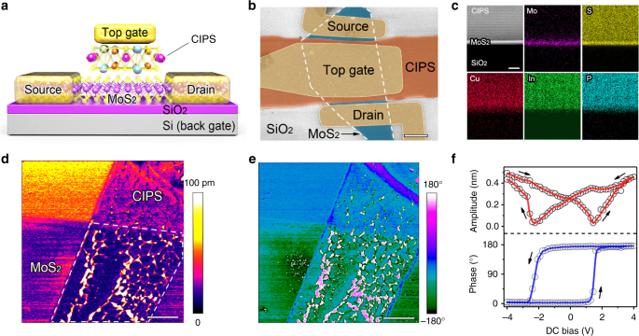2e . Fig. 1 CIPS/MoS2vdW heterostructure and NC-FET.a,bSchematic diagram (a) and False-color SEM image (b) of a CIPS/MoS2vdW NC-FET. Scale bar, 2 μm.cCross-sectional high-resolution TEM image of a vertically stacked CIPS/MoS2heterostructure on SiO2/Si substrate and corresponding EDS elemental map showing the distribution of Mo, S, Cu, In, and P. Scale bar, 5 nm.d,ePFM amplitude (d) and phase (e) of a CIPS/MoS2vdW heterostructure. The CIPS/MoS2stacked region is enclosed by dashed lines in (d). Scale bar, 2 μm.fThe off-field PFM amplitude (top) and phase (bottom) hysteresis loops during the switching process for CIPS flake The average SS during reverse sweep is less than 60 mV dec −1 for over seven decades of drain current, which is three orders of magnitude greater than that of TMD NC-FETs with bulk ferroelectric [15] , [16] , [17] (Supplementary Table 1 ). The great transistor performance can be attributed to the strong NC effect due to the trap-free CIPS/MoS 2 interface in vdW NC-FET. As the thickness of CIPS decreases, its drain current range for SS <60 mV dec −1 (over five decades for 15.4 nm CIPS and less than one decade for 13.3 nm CIPS) deteriorates. Nevertheless, the hysteresis of vdW NC-FET with a 13.3 nm CIPS is suppressed to a negligible value (3.4 mV) while the minimum SS (20.6 mV dec −1 for forward sweep and 48.6 mV dec −1 for reverse sweep) are still less than the thermionic limit. The effect of CIPS thickness on hysteresis and SS can be explained by the size effects on ferroelectricity of CIPS [30] and capacitance matching between C CIPS and C int . Thinning CIPS leads to a decrease in the remnant ferroelectric polarization, the steepness and width of the hysteresis loops, as shown in Supplementary Fig. 17 , resulting in a larger SS and smaller hysteresis. Moreover, | C CIPS | increases with decreasing the thickness of CIPS, leading to a small gate-voltage amplification A V and approaching to the hysteresis-free condition for NC-FET (| C CIPS | > C int ). More than 28 vdW NC-FETs on SiO 2 /Si substrate have been successfully fabricated with CIPS thickness from 13 to 80 nm, and CIPS thickness dependence of SS and hysteresis are summarized in Fig. 2i . Most devices (21 devices) exhibit SS < 60 mV dec −1 at room temperature and the main trend of measured SS is captured well by our model simulations (details are provided in Supplementary Note 4 and Supplementary Figure 18 – 23 ). According to the simulation results, the design space for sub-60 mV dec −1 SS and hysteresis-free operation in a vdW NC-FET gated by a CIPS layer is limited to t CIPS < 21 nm, and the SS can only be designed to 57 mV dec −1 to avoid hysteresis. In order to further optimize the performance of NC-FET, thin h-BN layers were integrated to the top-gate stack for capacitance matching and gate leakage current reduction, as illustrated in Fig. 3a . From the simplified equivalent capacitance network in Fig. 3b , incorporating a 7.5 nm BN layer (see Supplementary Fig. 24 for atomic force microscopy (AFM) characterization) into the top-gate stack can improve the capacitance matching between CIPS and underlying 2D FET by reducing C int , and thus leading to a suppression of hysteresis from 607 to 98 mV and negligible degradation of SS for reverse sweep, as shown in Fig. 3c, d , respectively. At the same time, the gate leakage current is reduced by more than 3 orders as shown in Fig. 3e . The design space for vdW NC-FET with BN interfacial layer was also explored using our compact model. The color area represents the design space for vdW NC-FET with non-hysteresis and sub-60 mV dec −1 SS. Obviously, the design space is considerably enlarged by integrating the thin BN into the gate stack. The simulation results show a hysteresis-free characteristic for vdW NC-FET with 7.5 nm BN and 48 nm CIPS, while a hysteresis of 98 mV is observed in Fig. 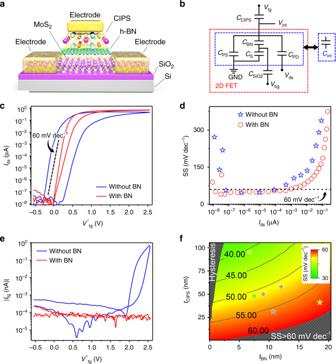Fig. 3 Electric characterization of CIPS/BN/MoS2vdW NC-FETs.a,bSchematic diagram (a) and equivalent capacitor network (b) of a CIPS/BN/MoS2vdW NC-FET.cTop-gate transfer characteristics of vdW NC-FETs with and without interfacial h-BN layer.V*tg=Vtg−Vth. Thickness of CIPS in CIPS/MoS2NC-FET is 49 nm and in CIPS/BN/MoS2NC-FET is 48 nm. The thickness of BN layer is 7.5 nm.d,eTop-gate SS−Idscharacteristics for reverse sweep (d) and leakage current (e) of CIPS/MoS2and CIPS/BN/MoS2vdW NC-FETs.fContour plot of simulated SS as a function of thickness of CIPS (tCIPS) and BN layer (tBN) atVds= 0.5 V andVbg= 0 V. Symbol, experimental data 3c . The deviation between experimental and model results can be explained by the non-uniformity in potential and charge at the CIPS/BN interface due to the absence of interfacial metal layer in the real device [31] . Fig. 3 Electric characterization of CIPS/BN/MoS 2 vdW NC-FETs. a , b Schematic diagram ( a ) and equivalent capacitor network ( b ) of a CIPS/BN/MoS 2 vdW NC-FET. c Top-gate transfer characteristics of vdW NC-FETs with and without interfacial h-BN layer. V * tg = V tg − V th . Thickness of CIPS in CIPS/MoS 2 NC-FET is 49 nm and in CIPS/BN/MoS 2 NC-FET is 48 nm. The thickness of BN layer is 7.5 nm. d , e Top-gate SS− I ds characteristics for reverse sweep ( d ) and leakage current ( e ) of CIPS/MoS 2 and CIPS/BN/MoS 2 vdW NC-FETs. f Contour plot of simulated SS as a function of thickness of CIPS ( t CIPS ) and BN layer ( t BN ) at V ds = 0.5 V and V bg = 0 V. Symbol, experimental data Full size image VdW NC-FET inverters A logic inverter was fabricated to evaluate the feasibility of vdW NC-FET for low-power applications. As shown in the schematic (Fig. 4a, b ), the logic inverter was constructed with two CIPS/MoS 2 vdW NC-FETs connected in series, serving as the pull-up load and pull-down driver, respectively. The pull-up load was realized by directly connecting the top gate of a NC-FET to the common source electrode. A typical vdW NC-FET inverter with W / L = 5.4/4.0 for load NC-FET and W / L = 2.4/5.5 for driver NC-FET, is shown in the false-color SEM image of Fig. 4c , where W and L denote the width and length of the transistor channels, respectively. 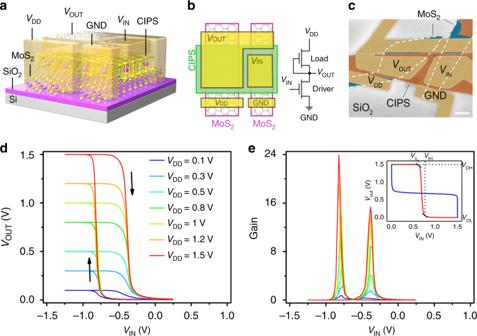Fig. 4 Electrical performance of vdW NC-FET inverter.a–cSchematic structure (a), circuit schematic (b) and false-color SEM image (c) of a vdW NC-FET inverter.W/L= 5.4/4.0 for load NC-FET andW/L= 2.4/5.5 for driver NC-FET. The thickness of CIPS flake is 42 nm. Scale bar, 2 μm.dRoom temperature voltage transfer characteristics,VOUT−VIN, of the logic inverter measured at variousVDD.eVoltage gain of the inverter at variousVDD. Inset: Noise margins of vdW NC-FET inverter atVDD= 1.5 V Figure 4d presents the voltage transfer curves, plot of input ( V IN ) versus output voltage ( V OUT ), of vdW NC-FET inverter under various supply voltages ( V DD ). Signal inversions are clearly observed with high V OUT at low V IN even though the V DD is down to 0.1 V for both forward and reverse sweeps. Comparing the V OUT versus V IN , a maximum voltage gain as ∼ 24 can be obtained for V DD = 1.5 V, which is considerably higher in comparison with TMDs based MOS inverters [32] , [33] , [34] . The noise margins of the inverter, NM L = 0.406 V DD and NM H = 0.493 V DD ((see Supplementary Note 5 and Supplementary Fig. 25 for determination of the noise margins), approach the idea noise margin (0.5 V DD ), indicating that the vdW NC-FET inverter is highly immune to electrical noise from the environment and very desirable for integration into multi-stage logic circuits, despite a hysteresis of 380 mV induced by the poor capacitance matching and the intrinsic negative-differential-resistance effect in NC-FET. Fig. 4 Electrical performance of vdW NC-FET inverter. a–c Schematic structure ( a ), circuit schematic ( b ) and false-color SEM image ( c ) of a vdW NC-FET inverter. W / L = 5.4/4.0 for load NC-FET and W / L = 2.4/5.5 for driver NC-FET. The thickness of CIPS flake is 42 nm. Scale bar, 2 μm. d Room temperature voltage transfer characteristics, V OUT − V IN , of the logic inverter measured at various V DD . e Voltage gain of the inverter at various V DD . Inset: Noise margins of vdW NC-FET inverter at V DD = 1.5 V Full size image VdW NC-FETs on flexible substrate A wide range of flexible electronic devices are typically powered by energy harvesting sources, it is necessary to demonstrate the scalability of vdW NC-FETs in flexible electronic applications to minimize the energy consumption. The layered structures of CIPS and TMDs offer a good mechanical flexibility for vdW NC-FET. 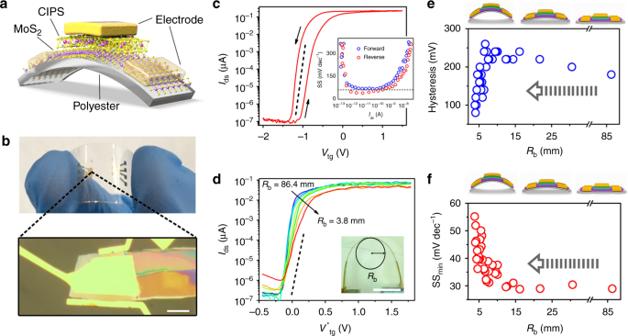Fig. 5 VdW NC-FETs on flexible substrate.a,bSchematic structure (a) and photograph (b) of a CIPS/MoS2vdW NC-FET on a flexible polyester substrate. The thickness of CIPS flake is 86.4 nm. Scale bar, 10 μm.cIds−Vtgcharacteristics of a flexible vdW NC-FET.Vds= 0.5 V. Inset, SS−Idscharacteristics.dTransfer characteristics of a flexible vdW NC-FET measured at the bending states withRbvalues of 86.4, 12.4, 7.5, 5.8, 4.8, 4.2, and 3.8 mm.V*tg=Vtg-Vth. Inset, photograph of a vdW NC-FET on stressed polyester substrate. Scale bar, 5 mm.e,fThe effect of bending radius on the hysteresis width (e) and SS (f) of the vdW NC-FET Figure 5a, b shows the structure and photograph of a flexible MoS 2 NC-FET with a pure CIPS dielectric layer atop a 130 um thick polyester substrate, respectively. The vdW NC-FET on flexible substrate exhibits a similar performance with an anticlockwise hysteresis loop and sustained sub-60 mV dec −1 switching, as shown in Fig. 5c (see Supplementary Figs. 26 and 27 for more vdW NC-FETs on flexible substrate). In order to investigate the stability of the device performance under static tensile strain, electrical characteristics were recorded with flexible NC-FETs under various bending curvature radius. Figure 5d presents the transfer characteristics of a vdW NC-FET measured at tensile bending states with bending radius ( R b ) from 86.4 to 3.8 mm (see Supplementary Note 6 and Supplementary Figure 28 for determination of bending radius). The steep switching characteristic with the minimum SS less than 60 mV dec −1 was preserved even with R b down to 3.8 mm, less than minimum bending radius reported in previous organic ferroelectric devices [35] . The slight decrease in on-state current with decreasing R b arises from the tensile strain induced polarization decrease in CIPS, while the increase in off-state current may result from the piezotronic effect of CIPS induced gate leakage current increase [23] , and I tg – V tg characteristics at various bending states are provided in Supplementary Fig. 29 . Surprisingly, the hysteresis window of the flexible vdW NC-FET was suppressed to 80 mV as the bending radius decreases to 4 mm, as shown in Fig. 5e , which is most likely due to the reduction of coercive field for stressed CIPS [36] . This conclusion is also supported by the thickness dependence of hysteresis shown in Fig. 2i and Supplementary Fig. 27 , where vdW NC-FETs on flexible substrate show relatively smaller hysteresis compared to devices on SiO 2 /Si substrate due to the residual stresses introduced during device fabrication. Figure 5f illustrates the extracted minimum SS of the device as a function of the bending radius. Sub-30 mV dec −1 SS can be achieved at the initial states with bending radius larger than 12 mm following a slight degradation of SS as R b decreases below 10 mm, which may result from the suppressed ferroelectric polarization due to the electrical breakdown under extreme bending condition [37] . However, it is clearly that all SS min values are better than the thermionic limit until the bending radius reaches 3.8 mm. Bending cycle test was also carried out with another device and sub-60 mV dec −1 switching characteristics were maintained up to 500 cycles (Supplementary Note 6 and Supplementary Fig. 30 ). The successful demonstration of flexible NC-FET with vdW ferroelectric and semiconductor represents a strategy to meet the ultralow-power operation in the emerging wearable computing applications. Fig. 5 VdW NC-FETs on flexible substrate. a , b Schematic structure ( a ) and photograph ( b ) of a CIPS/MoS 2 vdW NC-FET on a flexible polyester substrate. The thickness of CIPS flake is 86.4 nm. Scale bar, 10 μm. c I ds − V tg characteristics of a flexible vdW NC-FET. V ds = 0.5 V. Inset, SS− I ds characteristics. d Transfer characteristics of a flexible vdW NC-FET measured at the bending states with R b values of 86.4, 12.4, 7.5, 5.8, 4.8, 4.2, and 3.8 mm. V * tg = V tg - V th . Inset, photograph of a vdW NC-FET on stressed polyester substrate. Scale bar, 5 mm. e , f The effect of bending radius on the hysteresis width ( e ) and SS ( f ) of the vdW NC-FET Full size image In conclusion, NC-FETs have been successfully demonstrated using van der Waals ferroelectrics and TMDs. The adaptation to vdW layered semiconductor and ferroelectric enables the NC-FET with high performance, originating from the clean interface between MoS 2 and CIPS, and high bendability. The sub-thermionic switching characteristics and the observed drain-induced-barrier-rising effect and negative-differential-resistance characteristics have been confirmed to be the results of NC effect of CIPS. Hysteresis is considerably reduced by integrating a thin h-BN layer to the gate stack and negligible hysteresis is achieved in vdW NC-FETs with the thickness of CIPS less than 20 nm. Moreover, high-gain inverter based on vdW NC-FET is built. Sub-60 mV dec −1 SS can be retained and hysteresis alleviated for vdW NC-FETs on flexible substrate under a bending radius down to 3.8 mm. Our work demonstrates that NC-FETs with vdW ferroelectrics and TMDs are a promising architecture for low-power and wearable applications. VdW NC-FET device fabrication High-quality single crystals of CIPS, MoS 2 , and WSe 2 were synthesized by solid state reaction. The 2D flakes were all achieved by mechanical exfoliation from bulk crystals onto heavily doped silicon substrates with a 285 nm SiO 2 layer. TMD/CIPS and TMD/BN/CIPS heterostructures were produced with a dry transfer technique as reported. Cr/Au (5 nm/80 nm) electrodes were defined using standard e-beam lithography (EBL) process followed by metal thermal evaporation and lift-off process. Ten-nanometers Au film was used as a discharge layer for EBL processes on polyester substrate. Characterizations Layer number of MoS 2 and WSe 2 were identified by optical microscopy and micro-Raman spectroscopy (Witec) with a 532 nm laser. Atomic force microscopy (AFM, Bruker Dimension Icon or Asylum Research Cypher S) in a tapping mode was used to characterize the morphology of the CIPS and device. PFM measurements were carried out on a commercial atomic force microscope (Asylum Research Cypher S) under DART mode. Off-field hysteresis loops were obtained by recording the piezoresponse amplitude and phase 1 signals after individual DC bias was turned off. Electrical transport properties of vdW NC-FETs on SiO 2 /Si substrate were measured with an Agilent B1500A Semiconductor Device Parameter Analyzer in a vacuum chamber of 10 −2 torr. For the bending test, a micro translation stage was used to hold the flexible substrate on both sides and a manual handle to vary the distance between the two ends of the flexible substrate to control the bending curvature. Bending radius was estimated from the optical image of the strained substrate. The electrical properties of flexible NC-FETs at different bending states were recorded with Agilent B1500A in an air environment. Simulation A vdW NC-FET was treated as an underlying 2D FET in series with a ferroelectric capacitor. The transfer characteristics of 2D FET were obtained by solving the Poisson and drift-diffusion equation. Steady-state Landau-Khalatnikov equation was employed to model ferroelectric CIPS capacitor.